Genome sequence of the date palmPhoenix dactyliferaL Date palm ( Phoenix dactylifera L.) is a cultivated woody plant species with agricultural and economic importance. Here we report a genome assembly for an elite variety ( Khalas ), which is 605.4 Mb in size and covers >90% of the genome (~671 Mb) and >96% of its genes (~41,660 genes). Genomic sequence analysis demonstrates that P. dactylifera experienced a clear genome-wide duplication after either ancient whole genome duplications or massive segmental duplications. Genetic diversity analysis indicates that its stress resistance and sugar metabolism-related genes tend to be enriched in the chromosomal regions where the density of single-nucleotide polymorphisms is relatively low. Using transcriptomic data, we also illustrate the date palm’s unique sugar metabolism that underlies fruit development and ripening. Our large-scale genomic and transcriptomic data pave the way for further genomic studies not only on P. dactylifera but also other Arecaceae plants. The economic importance of the palm family plants (Arecaceae or Palmae) is second only to the grass family (Poaceae) among monocotyledons and the third among all plant families after legume (Leguminosae). Among the palm crops, the top three out of the five major domesticated palm species in the world are African oil palm ( Elaeis guineensis ), coconut ( Cocos nucifera ) and date palm ( Phoenix dactylifera )—the other two are peach palm ( Bactris gasipaes ) and betel palm ( Areca catechu ) (FAO, http://www.fao.org ). The economic utility of these palms are multifold, including staple food, beverages, ornamentals, building wood, and industrial materials [1] . P. dactylifera is a strict dioecious evergreen tree capable of living over 100 productive years. It is not only one of the oldest domesticated trees but also of socio-economic importance [2] . The earliest cultivation of P. dactylifera was recorded in 3,700 BC in the area between the Euphrates and the Nile Rivers [3] . It is thought to be native to the Arabian Peninsula regions, possibly originating from what is now southern Iraq. At a very early time, date palm was introduced by humans to northern India, North Africa, and southern Spain and it has a major economic role in the arid zones [4] . Saudi Arabia, one of the most important countries for date palm cultivation, has >10% of the world’s date palm trees (14% of the date production) and nearly 340 of ~2,000 varieties recorded around the world are grown here [5] . There have been a very limited number of genome-wide studies on P. dactylifera . One is a recent report on a draft genome assembly based on data generated from the Illumina GAII sequencing platform by a research team in Qatar [6] . They estimated the genome size (658 Mb), assembled 58% of the genome (382 Mb) and predicted 25,059 genes. Another is a comparative transcriptomic study on mesocarps of both oil and date palms based on pyrosequencing data from the Roche GS FLX Titanium platform [7] . Our effort on P. dactylifera genomics was launched in August 2008 and has delivered full-genome assemblies of its two organelles (158,462 and 715,001 bp for plastid [8] and mitochondrion [9] , respectively). We also constructed transcriptomic profiles for fruit development based on pyrosequencing data [10] . Here, we report our analyses of a more complete P. dactylifera genome assembly in comparison with three other selected varieties, as well as transcriptomic studies on genes related to abiotic resistance and fruit development. The study paves a way for further biological studies on P. dactylifera and comparative genomics for other palm family plants. Genome assembly and validation Our core data for contig assembly is composed of 31.4 million high-quality pyrosequencing reads generated from four fragment libraries of the Khalas variety, which cover 17.3 × of the estimated genome length (671.2 Mb, Supplementary Note 1 ) and were assembled into 194,980 contigs (N50=5,806 bp, 507.9 Mb). We further improved the continuity of the Newbler-assembled contigs using SOLiD reads from long mate-pair (LMP) libraries with variable insert sizes (nine libraries and 1–8 kb in length) and mapped ~73.9-Gb sequences uniquely to the contigs (122.1 × ). This intermediate built is composed of 82,863 contigs (N50=195.4 kb; 553.3 Mb). 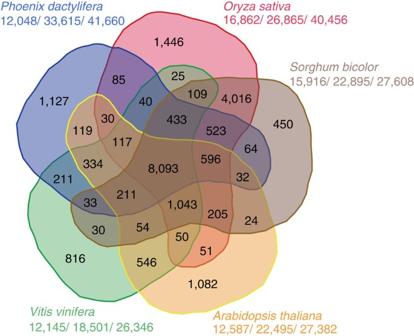Figure 1: A Venn diagram showing the distribution of shared gene families among representative angiosperms. Phoenix dactylifera,Arabidopsis thaliana,Oryza sativa,Sorghum bicolorandVitis vinifera(OrthoMCL 2.0.2,E<1e-5). The number of gene families, the number of genes in the families and the total number of genes are indicated under species names, which are separated by slashes. A total of 12,624 sequences in 1,127 gene families are unique toP. dactylifera,and these unique gene families are mostly related to DNA/RNA metabolic process and ion binding (Supplementary Table S15). The final assembly was extended based on BAC-end sequences, which contains 82,354 scaffolds (N50=329.9 kb; 558.0 Mb) ( Table 1 and Supplementary Table S1 ). On the basis of our estimated genome size, this assembly (605.4 Mb) covers 90.2% of the genome when contigs <500 bp are also taken into account. Table 1 An overview of the Phoenix dactylifera genome assembly. Full size table To assess the coverage and completeness of the genome assembly, we used assembled sequences from 10 BACs (variety Khalas ) and six fosmids (from a northern African variety Deglet Noor ) ( Supplementary Table S2 ). The alignments are unambiguous—98.5% and 96.5% for the BACs and the fosmids, respectively—and high-quality with no misalignment ( Supplementary Figs S1 and S2 ). We also validated the assembly using ESTs from our own transcriptomic projects [11] , the Qatar [6] and the CNRS (Centre National de la Recherche Scientifique) group [7] , and found that 96.3%, 90.8% and 96.4% of the EST datasets are matched to the genome assembly, respectively. The reasons for the variable matching rates are largely platform-dependent, such as short read length and variable error rates ( Supplementary Table S3 ). Genome annotation We built a much larger pool of gene models for P. dactylifera than those previously reported, by combining ab initio predictions (Fgenesh++ [12] ), EST assemblies (pyrosequencing data), RNA-seq reads (SOLiD data), plant protein-coding genes and protein domain information for gene annotation. The effort yielded 41,660 gene models (42,957 isoforms) in 10,363 scaffolds (472,329,057 bp in length; 84.6% of the total length) ( Supplementary Note 2 , Supplementary Table S4 and Supplementary Fig. S3 ). Our proteome comparison of P. dactylifera to Arabidopsis thaliana , Oryza sativa , Sorghum bicolor and Vitis vinifera revealed that 8,093 gene families are shared among all five plant genomes and 1,127 gene families are unique to P. dactylifera ( Fig. 1 ). Figure 1: A Venn diagram showing the distribution of shared gene families among representative angiosperms. Phoenix dactylifera , Arabidopsis thaliana , Oryza sativa , Sorghum bicolor and Vitis vinifera (OrthoMCL 2.0.2, E <1e-5). The number of gene families, the number of genes in the families and the total number of genes are indicated under species names, which are separated by slashes. A total of 12,624 sequences in 1,127 gene families are unique to P. dactylifera, and these unique gene families are mostly related to DNA/RNA metabolic process and ion binding ( Supplementary Table S15 ). Full size image There are two types of repetitive sequences in any given plant genomes: mathematically-defined and biologically-defined repeats [13] , [14] . In P. dactylifera , most biologically-defined repeats are retrotransposons, accounted for 21.99% of the genome, of which 14.03% and 4.17% are Ty1/Copia and Ty3/Gypsy, respectively. Annotated non-LTR retrotransposon LINEs and DNA transposons (hAT/Ac, CACTA/EnSpm and MITEs) make up merely 0.96% of the genome. Aside from ~2.15% microsatellite-derived mathematically-defined repeats ( Supplementary Table S5 ), the P. dactylifera genome harbours 38.41% repetitive sequences ( Supplementary Table S6 ), a proportion that is within the range of other sequenced plant genomes, including O. sativa (39.5%), V. vinifera (41.4%) and P. trichocarpa (42%). Relying on the relative completeness of our genome assembly, we discovered Ty1/Copia has a much higher copy number than Ty3/Gypsy but in most other sequenced plant genomes the former has been found to be always less in number than the latter. Further analysis based on our in-house generated data from other palms confirmed that the pattern holds true for all palm family plants ( Supplementary Table S7 ). The most abundant Ty1/Copia elements in P. dactylifera show the highest homology to the rice retrotransposon element 1 (ref. 15 ) in the conserved region of the reverse transcriptase genes. Genome-wide duplication Genome-wide duplication (GWD) is rather prevalent among angiosperms that share the same ancestor ~150 Mya (refs 16 , 17 ). GWD provides essential genetic material for the creation of novel functions for adapting new environment and tolerating biotic and abiotic stresses [18] . Using 4,215 paralogous gene pairs in 411 collinear regions of the P. dactylifera genome assembly, we assessed the distribution of Ks or 4DTv to show two distinct peaks: Ks ~0.314 (4DTv~0.107) and Ks ~0.833 (4DTv~0.332) ( Supplementary Fig. S4 ). After the exclusion of the recent GWD of Z. mays genome, the curve is similar to that of P. trichocarpa but not to those of Gramineae plants ( Fig. 2 ); the first peak corresponds to a GWD event shared among all angiosperms and the second peak derives from either a single more ancient GWD or massive consecutive segmental duplications when the slow substitution rate of the palm family [19] and abundant fossil records from ~90 Mya (ref. 20 ) are both considered ( Supplementary Note 3 ). We also found significant macro-synteny between P. dactylifera and other monocotyledons ( Supplementary Fig. S5 ) but failed to observe it between P. dactylifera and any dicotyledons. Remarkably, the biggest scaffold, pdS00001 (~4.5 Mb in length), appears highly conserved and is part of the ‘concentric circles’ of monocotyledons [21] ( Fig. 3 ). 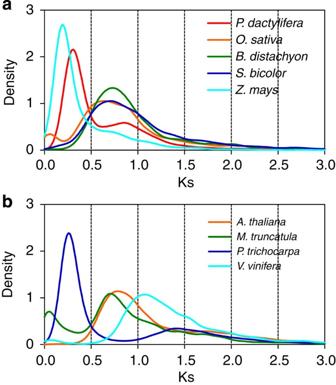Figure 2: Ks distribution of GWD in selected monocotyledons and dicotyledons. The density distribution of each monocotyledon (a) or dicotyledon (b) was calculated based on kernel density estimation with a bin size of 0.001. The evolutionary rate is relative slow in trees47,48, such as those ofP. trichocarpaandV. vinifera. We suppose that theP. dactyliferagenome also has this character similar to oil palm7. The minor peak ofO. sativa(Ks ~0.06) was recently suggested to be a GWD event happened ~70 Mya and the genome underwent an illegitimate recombination followed by fast evolution49.Z. mayshad a recent GWD event (Ks~0.2, ~5–12 Mya) as compared with other Gramineae species50. InM. truncatula, a peak near 0 (Ks~0.05) is due to local duplication and faster evolution rate as compared with other vascular plants51. Figure 2: Ks distribution of GWD in selected monocotyledons and dicotyledons. The density distribution of each monocotyledon ( a ) or dicotyledon ( b ) was calculated based on kernel density estimation with a bin size of 0.001. The evolutionary rate is relative slow in trees [47] , [48] , such as those of P. trichocarpa and V. vinifera . We suppose that the P. dactylifera genome also has this character similar to oil palm [7] . The minor peak of O. sativa (Ks ~0.06) was recently suggested to be a GWD event happened ~70 Mya and the genome underwent an illegitimate recombination followed by fast evolution [49] . Z. mays had a recent GWD event (Ks~0.2, ~5–12 Mya) as compared with other Gramineae species [50] . In M. truncatula , a peak near 0 (Ks~0.05) is due to local duplication and faster evolution rate as compared with other vascular plants [51] . 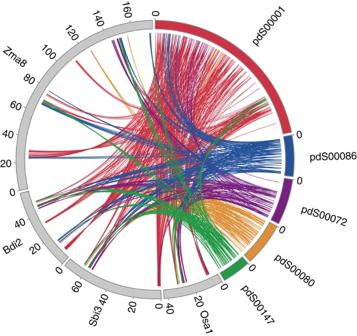Figure 3: Macro-synteny amongP. dactyliferascaffolds and other monocotyledon chromosomes. Scaffolds pdS00001 (4.5 M), pdS00072 (1.1 M), pdS00080 (1 M) pdS00086 (1 M) and pdS00147 (0.7 M) have the same syntenic pattern with other monocotyledons. In addition, the latter four scaffolds have syntenic regions with pdS00001 and are inferred to be duplicated at monocotyledon ancestry (Supplementary Fig. S5). The unit of scale is million base pairs or Mb for other monocotyledon chromosomes. AllP. dactyliferascaffolds are enlarged 30 × for illustration. Full size image Figure 3: Macro-synteny among P. dactylifera scaffolds and other monocotyledon chromosomes. Scaffolds pdS00001 (4.5 M), pdS00072 (1.1 M), pdS00080 (1 M) pdS00086 (1 M) and pdS00147 (0.7 M) have the same syntenic pattern with other monocotyledons. In addition, the latter four scaffolds have syntenic regions with pdS00001 and are inferred to be duplicated at monocotyledon ancestry ( Supplementary Fig. S5 ). The unit of scale is million base pairs or Mb for other monocotyledon chromosomes. All P. dactylifera scaffolds are enlarged 30 × for illustration. Full size image Expansion of the late embryogenesis abundant family Date palms thrive in arid regions of the Middle East and North Africa, armed with its resistances to abiotic stresses, including drought, salinity and heat. Despite possible roles of physiological mechanisms, expansion of resistance-related gene families in P. dactylifera is expected. We scrutinized the late embryogenesis abundant (LEA) gene family that has been classified into eight groups and 84 gene members across taxa ( Supplementary Table S8 ). The group 2 LEA (or LEA2) genes are of particular abundance in the P. dactylifera genome assembly; there are 62 LEA2 members in P. dactylifera , as compared with 52 and 46 in rice and sorghum, respectively. Corresponding to their individual member expansions, this P. dactylifera LEA family also shows a complex expression profile in different tissues/organs and developmental stages according to our transcriptomic data. Among 12 different samples, 67 LEA genes were detected as expressed, most of them in a tissue-/organ-specific manner ( Fig. 4 ). In general, the subfamilies of LEA1, LEA3, LEA4, LEA5, LEA6, SMP and Dehydrin are seed associated or male flower associated, whereas the LEA2 members are nearly all ubiquitous. As some of the LEA genes have been demonstrated to enhance tolerances to desiccation, cold, salination and osmosis stresses in various plants [22] , expansion of the P. dactylifera LEA2 may be responsible, at least in part, for the resistance to abiotic stresses. 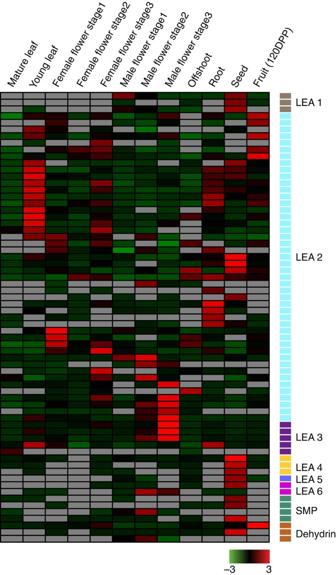Figure 4: Expression patterns of the LEA genes among 12 tissues ofP. dactylifera. The LEA subfamilies are colour-coded (on the right side). The expression levels are normalized based on theZ-score method (scale bar) over all libraries (on the top). Figure 4: Expression patterns of the LEA genes among 12 tissues of P. dactylifera . The LEA subfamilies are colour-coded (on the right side). The expression levels are normalized based on the Z -score method (scale bar) over all libraries (on the top). Full size image Defining differentially expressed genes Since fruit or date is the most economically valuable product of date palm, we made an effort to identify differentially expressed genes (DEGs) involved in fruit development and ripening to provide a starting point for further investigation. We identified 4,134 DEGs, whose expressions significantly vary among seven fruit developmental stages, using RNA-Seq data; ( Supplementary Table S9 and Supplementary Data 1 ). When clustering the DEGs into different groups (upregulated, downregulated, not-regulated group 1 and not-regulated group 2; Supplementary Fig. S6 ), we found that the two major groups, the up-regulated and the downregulated, show different enrichments of DEGs—gluconeogenesis, cellular carbohydrate metabolism and small molecule biosynthesis in the upregulated group as opposed to biological regulation, transcription and regulation of RNA metabolic process in the downregulated group (hypergeometric P <0.01, Bonferroni false discovery rate <0.05; Supplementary Tables S10 and S11 ). This result indicates that most of the molecular events are down-regulated in the late stage of fruit development except sugar accumulation resulting in unusually high sugar content in dates. Kyoto encyclopedia of genes and genomes pathways Our analyses on transcriptomic data were focused on fruiting based on Kyoto Encyclopedia of Genes and Genomes (KEGG) pathways. It is unequivocal that ‘carbohydrate metabolism’ is the most activated pathway at every single stage of the fruit development and ripening. ‘Energy metabolism’ and ‘metabolism of other amino acids’ are the second and the third highly expressed pathways, respectively ( Supplementary Fig. S7a ). Within the ‘carbohydrate metabolism’ pathway, we observed that genes directly associated with sugar metabolism are much more activated at the later stages of fruiting and that their expressions peak at 120 or 135 days post pollination (DPP) ( Supplementary Fig. S7b ). Taking the ‘fructose and mannose metabolism pathway’ as an example, the gene expression of this pathway increases gradually and reaches its highest level at 120 DPP. This general pattern provides a possible explanation for the high fructose content in the dates. Many of the ‘energy metabolism’-related genes are also elevated at the later stages, similar to that in ‘carbohydrate metabolism’ ( Supplementary Fig. S7c ). However, genes involved in photosynthesis are highly activated at the middle of the fruit development (75 DPP), when fruits remain green and their sizes are close to those of the mature form. Sugar metabolism As dates are famed for their high sugar content, we constructed gene expression profiles of 30 sugar metabolic enzymes and clustered them into two essential groups: early expressed genes and late expressed genes ( Fig. 5a and Supplementary Data 2 ). We first compared gene expression between fruit and leaf, and noticed that ribulose-1,5-bisphosphate carboxylase and two other enzymes genes, pyruvate orthophosphate dikinase and fructose-1, 6-bisphosphatase I, which are involved in invertible catalyzed sucrose synthesis reaction, are expressed much higher in green leaves. This result indicates that most of the sucrose accumulation in fruit may be contributed from leaves. C4-carbon fixation enzyme, phosphoenolpyruvate carboxylase, appears upregulated gradually during fruiting, perhaps having an important role in supplying carbon source at the late fruiting stages. Most other carbon assimilation-associated genes show a similar pattern where higher expression is observed in fruits rather than in green leaves and this also holds true in oil palm [7] ( Fig. 5a and Supplementary Fig. S8 ). These results provide evidence that date palm fruit or the date is also involved in carbon fixation or refixation reaction during fruit development and produces pyruvate, glycerate-3-P and sucrose for both glycolysis and sugar accumulation. We also looked into sucrose metabolism and the expression profiles of its three key enzymes [23] , [24] : sucrose synthase, sucrose-phosphate synthase and invertase ( Fig. 5a ). The transcriptions of sps and inv , not sus , show higher levels at the late stage, which agree with a previous observation on sugar content in date palm [25] and the key role assigned to sucrose-phosphate synthase, observed in citrus [26] , sugarcane [27] and banana [28] . The increasing expression of inv also supports the mechanism where invertase splits sucrose into glucose and fructose, leading to the final fructose deposition in dates. Of particular interest is the notion that starch hydrolysis and carbon fixation pathways are both switched on, and related genes are highly expressed at 120 DPP. These two pathways also contribute to the glucose and fructose accumulation in dates ( Fig. 5b ). 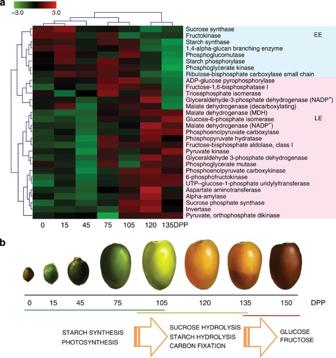Figure 5: Expression profiling of sugar metabolism-related genes at different fruiting stages. (a) Gene expression profiling of 30 key enzymes related to sugar metabolism. The hierarchical clustering shows that these genes can be classified into two patterns: genes expressed at the early developmental stages (EE, blue, 0–75 DPP) and at the late developmental stages (LE, red, 105–135 DPP). (b) Summary of sugar metabolisms during fruit development and ripening. Fruits at 150 DPP are completely ripe and we were unable to extract enough RNA for RNA-seq. Figure 5: Expression profiling of sugar metabolism-related genes at different fruiting stages. ( a ) Gene expression profiling of 30 key enzymes related to sugar metabolism. The hierarchical clustering shows that these genes can be classified into two patterns: genes expressed at the early developmental stages (EE, blue, 0–75 DPP) and at the late developmental stages (LE, red, 105–135 DPP). ( b ) Summary of sugar metabolisms during fruit development and ripening. Fruits at 150 DPP are completely ripe and we were unable to extract enough RNA for RNA-seq. Full size image Genetic diversity among varieties On genetic diversity, P. dactylifera is unique in several counts. First, it is a long-lived vegetatively propagated (offshoots are often used) species similar to poplar, having potential to contribute gametes to multiple generations in that a single genotype can persist in a garden for millennia. Second, a single phenotype, always female, can be selected as a clone to grow for further cultivation and selection. Third, the history of a date palm variety may be more complex than one anticipates—being carried for unusually long distance, cross-bred very intensively, and selected very heavily. As the Khalas genome assembly has an exceedingly high coverage of 122 × , we were able to define its allelic differences and calculated its single-nucleotide polymorphism (SNP) and indel densities as 2.57 and 0.10 per kb, respectively. We also identified the SNP (indel) densities for Agwa , Fahal and Skury , which are 6.10 (0.25), 5.51 (0.15) and 6.24 (0.20) per kb, respectively ( Supplementary Tables S12 and S13 ). Although sequence assemblies of seven other varieties are also publically available [6] , the genome coverage of these assemblies is rather low for short read-based sequence mapping, ranging from 12 × to 39 × . On the basis of our analysis, their SNP densities range from 3.85 per kb to 6.63 per kb, which are slightly higher than what expected but not very far off from the range of high-coverage assemblies. Chromosomal regions with reduced genetic diversity or ‘SNP deserts’ are often observed and linked to beneficial mutations that are often related to strong positive selection [29] . Over the past decade, several studies on SNP deserts have been reported in both mammals [30] , [31] and plants [32] , [33] , [34] , [35] , [36] . Our previous study found that agronomically important QTLs, such as MADS-box and the Waxy genes, are located in rice SNP deserts [32] . A detailed statistical analysis also revealed positive selections on functional genes and degenerative effects on gene expression in SNP deserts that are closely related to domestication [33] . It was reported that low-SNP regions or SNP deserts in the cultivated rice are presumably attributable to domestication processes that include artificial selection, population size reduction, introgression and selfing [34] , and thousands of candidate genes have also been identified for rice domestication [35] . On the basis of these discoveries, we investigated how selection has left its signatures in genomes of different date palm varieties by first evaluating the distribution of SNPs on large scaffolds and subsequently pinning down functional genes that are obviously selected, especially those closely involved in sugar and energy metabolisms. Clearly, SNPs/indels are not randomly distributed but exhibit a bimodal curve ( Fig. 6 ), where the low-SNP peak (<1 SNP per kb in a minimal length of 10 kb, about 18% of the genome assembly; Supplementary Fig. S9 and Supplementary Table S14 ) reflects trait selection in cultivation and thus considered as the signature of domestication, and this result is consistent with the previous reports in rice [32] , [33] , [34] , [35] . The SNP frequency distributions appear to have two different patterns among the varieties. The most popular commercial varieties, Khalas , Medjool and Deglet Noor , together with their backcrossed descendants, KhalsFx ( Khalas × Khalas F1), Medjool BC4 and Deglet Noor BC5, have a more obvious bimodal SNP distribution. In contrast, the distribution of non-commercial varieties AlrijalF and Fahal only have the major peak. Furthermore, the backcrossed descendants should have higher proportion of SNP desert regions as compared with their recurrent female parents ( Deglet Noor and Medjool ), as backcrossing is known to reduce genetic effect by one-half at each generation theoretically, and the reason why backcrossed P. dactylifera descendants are more conserved than their recurrent parents [6] may be related to both trait selection and artificial pollination (usually by hands and using commercial pollens with ambiguous origin). 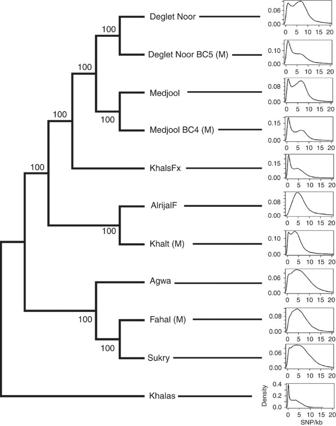Figure 6: Phylogenetic analysis of 11P. dactyliferavarieties based on SNPs and their SNPs frequency distributions. The phylogenetic tree was constructed by using all SNP sites of the varieties (NJ method with 1,000 bootstrap, MEGA 5.0). The series of plots show SNP density (SNP per kb, the horizontal axis) and frequencies (the vertical axis). SNP frequency was calculated based on a 10-kb sliding window in 1-kb steps. The modes of SNP distribution are compounding, where the minor mode is contributed by SNP deserts. Figure 6: Phylogenetic analysis of 11 P. dactylifera varieties based on SNPs and their SNPs frequency distributions. The phylogenetic tree was constructed by using all SNP sites of the varieties (NJ method with 1,000 bootstrap, MEGA 5.0). The series of plots show SNP density (SNP per kb, the horizontal axis) and frequencies (the vertical axis). SNP frequency was calculated based on a 10-kb sliding window in 1-kb steps. The modes of SNP distribution are compounding, where the minor mode is contributed by SNP deserts. Full size image As compared with that of the whole genome, the gene/repeat ratio of SNP deserts is over 3 × higher (3.12 versus 1.00; Pearson’s χ 2 value=13.541, P =0.000233). Non-synonymous SNPs are also enriched in SNP deserts (1.76 versus 1.18; Pearson’s χ 2 value=60.47, P =0). Furthermore, we also calculated gene density in SNP deserts and the whole genome by defining gene density as Ds gene per kb: 0.083 for SNP deserts (9,036 genes in 108,259 kb) and 0.069 for the genome average (41,660 genes in 605,351 kb). This result suggests that gene density is higher in SNP deserts as opposed to the genome average and it is further supported by the notion that there are also a higher proportion of gene families in SNP deserts. In addition, we found that SNP deserts tend to recruit genes associated with abiotic/disease resistances and energy/sugar metabolisms ( Table 2 ). Table 2 Genes and gene families enriched in SNP deserts. Full size table The extremely broad geographic distribution of P. dactylifera implies that it either has evolved as a plant covering extensive soil and climatic conditions or spreads with help from humans after having originated from a more limited geographic region. Owing to rather limited sampling, it is very difficult for us to draw a clear picture of the actual origin of date palm but we noticed that the northern African varieties, Deglet Noor and Medjool , are significantly diverged from the Middle Eastern varieties, as Saudi Arabian varieties ( Khalas , Agwa , Fahal and Sukry ) are clustered into a single clade ( Fig. 6 ). These results indicate that geographic isolation and artificial selection may both contribute to the diversity and evolution of P. dactylifera . Plant genomics is now entering a new era when genome assemblies are being produced based on complementary data from different platforms where high-coverage and satisfactory contiguity can both be achieved. Our initial analysis of the P. dactylifera genome provides a detailed view on genome-wide structural parameters of genes, histories of genome/gene duplications, genetic diversities of cultivar resources and functional genes in key functional categories. There are other important remaining issues for further exploitations. First, the current P. dactylifera genome assembly is much improved in both precision and contiguity, allowing us to position the genome in an evolutionary context by carrying out comparative studies between and among species and varieties. Second, because P. dactylifera is an obligate out-crossing species and its recessive alleles tend to be maintained in a heterozygous state, as we already observed in Khalas , more P. dactylifera varieties should be sequenced to a high coverage for quantitative trait mapping. Third, as we observed, the palm family seems to have a unique ratio of common retrotransposons so that it is desirable to classify and date them to investigate the possible reasons as to how repeats of different types may relate to genome dynamics, such as the generation of new genes. Fourth, high-quality sequence assemblies are of essence for better genome annotation for plants, as plant genomes are often large and structured very differently from animal genomes [37] . Fifth, many biological features unique to date palm or the palm family trees in general, such as fruit and nutrition content diversities, are to be studied in greater details at molecular levels, providing better knowledge for improving date quality and yield. Materials We collected P. dactylifera tissue samples (green leaves, yellow leaves, flowers, fruits, offshoots, and roots) for the following varieties: Khalas (female) and Fahal (male) samples from a date palm farm in Al-Hssa Oasis (25°04′35″N, 49°06′24″E), and Sukry (female) and Agwa (female) samples from Al-Qassim and Al-Medina Al-Monwarh, respectively, in Saudi Arabia. The fruit samples in various developmental stages of Khalas were harvested from a date palm farm at Al-Kharj (24°08′54″N, 47°18′18″E), Saudi Arabia. After thorough washing with double-distilled water, we immediately froze the samples in liquid nitrogen and transported them to the laboratory on dry ice. The samples were stored inside −80 °C freezers until use. DNA isolation Our DNA extraction protocol combines the high-molecular-weight DNA extraction [38] and hexadecyl trimethyl ammonium bromide (CTAB) method [39] for improved removal of polysaccharides and other contaminations. The date palm tissues were ground into a fine powder in the presence of liquid nitrogen and subsequently homogenized in HB buffer (10 mM Tris–HCl, 80 mM KCl, 10 mM EDTA, 1 mM spermidine, 0.5 mM spermine, 0.5% β-mercaptoethanol, 0.5 M Sucrose, pH 9.4). After several rounds of centrifugation at 800 × g to remove tissue residues, the nucleus-containing pellets were collected after centrifugation at 2,000 × g for 10 min. The nuclei were broken by osmotic pressure in CTAB lysis solution (2% CTAB, 1.4 M NaCl, 0.1 M Tris–HCl at pH 8.0, 0.02 M EDTA at pH 8.0) at 70 °C for 45 min. After a phenol–chloroform extraction, DNA samples were precipitated using precooled isopropanol and washed twice with 70% ethanol. RNA extraction Total RNA was extracted from 5 g of plant material by grinding it in liquid nitrogen and it was subsequently dissolved in 20 ml of preheated extraction buffer at 65 °C (ref. 40 ). The RNA sample was extracted twice with equal volumes of chloroform: isoamyl alcohol (24:1) in the presence of a 1/4 volume of 10 M LiCl and precipitated overnight at 4 °C. The RNA pellet was collected via ethanol precipitation and dissolved in 500 μl of SSTE (sodium dodecyl sulfate–Tris–HCl–EDTA) buffer. After futher extraction with equal volume of chloroform: isoamyl alcohol (24:1), the purified RNA was precipitated and treated with DNase I. Shotgun library construction and sequencing For Roche/454 data acquisition, 5 μg of genomic DNA was sheared into 500–800 bp fragments with a Nebulizer and both DNA ends were filled enzymatically. Library construction and the emPCR were performed according to the GS FLX Titanium General Library Preparation Guide and emPCR Method Manual (Roche), respectively. For the SOLiD data acquisition, 20 μg or more DNA (depending on insert size) samples were used to construct LMP libraries, according to the SOLiD 4 System Library Preparation Guide (Life Technologies), and the cDNA was sheared into fragments (1–8 kb) with hydroshear. After end-filling, the DNA fragments were ligated to the LMP adaptors and circularized. For RNA-seq, we used the RiboMinus Plant Kit for RNA-Seq (Life Technologies) to remove the ribosomal RNA from DNase I-treated total RNA. The starting material was 7 μg of total RNA, which yielded ~700 ng of RiboMinus RNA (rmRNA). Two hundred nanograms of rmRNA was used for the transcriptome library construction according to the SOLiD Total RNA-Seq Kit protocol. BAC DNA extraction and BAC-end sequencing The P. dactylifera BAC library was constructed (by Amplicon Express, Washington) with Hin dIII- and- Eco RI-digested DNA and the pCC1BAC vector (Epicentre). The quality of the library was assessed by using restriction digestion with Hin dIII of 28 randomly picked clones (116 kb to 131 kb). A total of 110,592 clones were randomly picked and stored in 384-well plates. For BAC-end sequencing, we extracted DNA from a 1 ml culture using an alkaline lysis protocol [41] in a 96-well filter plate (Thermo Fisher). Two micrograms of BAC DNA was used for the sequencing reaction with the BigDye Terminator v3.1 Cycle Sequencing Kit (Life Technologies). Genome assembly The backbone of our genome assembly was largely based on pyrosequencing reads. First, we assembled quality-filtered reads to build contigs using the default settings of Newbler (version 2.5.3). Second, we mapped the SOLiD mate-pair tags using BioScope (version 1.3) to the Newbler consensus contigs and estimated gap length according to insert sizes of the mate-pair libraries using a SOLiD-specific tool called HAPS (version 0.1.200; http://solidsoftwaretools.com/gf/project/haps/ ) with the linked read number ≥10. After filtering out short and repeat-containing contigs, we used the unique contigs (≥500 bp) to build super-contigs. Third, we filled gaps in the super-contigs by using both the Newbler contigs and pyrosequencing reads with a minimal 15-bp matched end. Finally, we used the BACs whose two end sequences were properly aligned to the super-contigs to construct the final scaffolds. The genome annotation files, mapping results of date palm varieties, mapping results of transcriptome data, and the assembled full-length cDNA sequences are available at the JCGR website ( http://www.kacst.edu.sa/en/depts/jcg/home/Pages/default.aspx ). LEA gene identification We searched LEA domains (Pfam with E value ≤1e-5) against the predicted P. dactylifera gene models and other sequenced plant genes/genomes using HMMER v3.0 and validated the candidate LEA genes using Blastp against plant LEA protein sequences of UniProt ( http://www.uniprot.org/ ). We aligned the SOLiD RNA-seq data (12 different tissues/organs and >40 million reads for each library) to the candidate LEA genes and the mapped read number was normalized based on the Z -score method for heatmap (heatmap2 of R package). Fruit-ripening-related gene expression We mapped the SOLiD RNA-Seq reads generated from P. dactylifera samples at seven distinct fruit developmental stages (0, 15, 30, 60, 90, 120 and 135 DPP) to the gene models using Bioscope v1.3 with default parameters. The uniquely mapped reads for gene expression were defined with a threshold of >5 and normalized to per kb of genes per million reads (RPKM) [42] . We annotated genes using InterProScan, KAAS (KAAS, http://www.genome.ad.jp/tools/kaas/ ) [43] and KEGG basic metabolic pathway. We identified DEGs during fruit ripening using edgeR [44] and clustered all them based on RPKM values using the R hclust function. We also conducted gene ontology enrichment analysis of the two major clusters using AGRIGO [45] . On the basis of gene annotation and transcriptome analysis, we estimated gene expression levels of each pathway in the KEGG ‘metabolism’ category according to the following protocol. First, expression levels for each KEGG ortholog (KO) were calculated as the sum of all RPKM values for each gene. This value at seven distinct fruit development stages was defined as the KO expression value. All KO expression values in a single pathway were then averaged, giving the pathway expression value. Finally, the average value of pathway expression values for each subcategory of the KEGG ‘metabolism’ category was calculated. Diversity analysis of date palm varieties We mapped the SOLiD mate-pair reads from Khalas , Agwa , Sukry and Fahal (male) to the our ( Khalas ) genome assembly and called sequence variations both between the two alleles of a genome and among all genomes using Pileup, a software package of SAM tool [46] . To reduce false positives, we filtered the SNPs and indels using total read coverage ≥4, frequency of SNPs or indels ≥20%, and observed SNPs or indels ≥2 as thresholds. We also used raw sequencing reads of AlrijalF , Deglet Noor , Deglet Noor BC5 , Khalt , KhalsFx , Medjool and Medjool BC4 from the SRA database for a combined analysis. Accession codes: Date palm genome assembly, BAC clones, and transcriptomic data were deposited in Genbank with BioProject ID PRJNA83433, and the EST raw reads were submitted to Sequence Read Archive (SRA; SRA045434 , SRA049307 and SRX096040 ). How to cite this article: Al-Mssallem, I. S. et al. Genome sequence of the date palm Phoenix dactylifera L. Nat. Commun. 4:2274 doi: 10.1038/ncomms3274 (2013).